Multistep kinetic self-assembly of DNA-coated colloids Equilibrium self-assembly relies on the relaxation of disordered mixtures of building blocks towards an ordered ground state. The main drawback of this traditional approach lies in the kinetic traps that often interrupt the progression of the system towards equilibrium and lead to the formation of arrested phases. The latest techniques to control colloidal interactions open up the possibility of exploiting the tendency to dynamically arrest in order to construct amorphous materials with a specific morphology and local separation between multiple components. Here we propose strategies to direct the gelation of two-component colloidal mixtures by sequentially activating selective interactions. We investigate morphological changes in the structure of the arrested phases both by means of molecular dynamics simulations and experimentally by using DNA-coated colloids. Our approach can be exploited to assemble multicomponent mesoporous materials with possible applications in hybrid photovoltaics, photonics and drug delivery. Self-assembly is traditionally regarded as the process through which an initially disordered mixture of mesoscopic particles relaxes towards an equilibrium ordered phase only driven by local interactions between its building blocks. Most often, the main issue in equilibration-based (equilibrium) self-assembly lies in the tendency of colloidal mixtures to undergo dynamic arrest and form metastable disordered phases: precursors of the crystalline ground state [1] , [2] , [3] . A fitting example is provided by DNA-coated colloids (DNACCs) that, owing to the specificity and programmability of the interactions, are considered as the ideal test bench for equilibrium self-assembly. Because of the strength and the sharp thermal activation of the interactions [4] , [5] , [6] , [7] , however, DNACCs reveal a strong tendency to kinetically arrest into amorphous structures. Crystallization has been reliably achieved only using nanoscale particles [7] , [8] , [9] , [10] , [11] , [12] , [13] , [14] , whose interactions are weaker and thermal activation smoother, whereas scaling up to slightly larger building blocks has turned out to be difficult [7] , [15] , [16] . Defining self-assembly as a mere equilibration process is very restrictive. Nature itself provides examples of amorphous, yet functional, materials assembled by controlling the kinetic arrest of out-of-equilibrium systems in their pathway towards the ground state [17] , [18] , [19] , [20] , [21] . This type of kinetic self-assembly is intrinsically more flexible and reliable than its equilibrium counterpart, allowing control over the morphology of the final phase by tuning both the interactions and the kinetic pathway leading to dynamic arrest [22] , [23] , [24] . In this article, we design and test two-component mixtures of colloidal particles with selective interactions, and control their dynamic arrest by activating different interactions at different stages of the kinetic self-assembly protocol. Specifically, one of the components is programmed to aggregate before the other, providing a template or a scaffold for the aggregation of the second. The binary mixtures are tested via both event-driven molecular dynamics (MD) simulations and experimentally using DNACCs. The sharp thermal activation of the interactions that makes DNACCs unsuitable for equilibrium self-assembly makes them ideal for the purpose of triggering specific interactions at well-defined stages of a quenching procedure. Exploiting this feature and the selectivity of the Watson–Crick base paring, we accurately replicate in-silico experiments and achieve an unprecedented control over the morphology of the target materials. In contrast to equilibrium self-assembly of DNACCs, only possible for nanoscale objects, our approach can be applied to the whole range of colloidal sizes. Moreover, we only rely on isotropic, yet selective and controllable [23] , [24] , interactions without the need of particle shaping [25] or directional bonds [26] , [27] , [28] . We propose two schemes that exemplify the potential of our strategy. For each example, we employ two different DNACC species, but similar criteria can be adopted to design arbitrarily complex systems with more than two components, more aggregation stages or modified interaction schemes. In the final section, we describe some of the expected technological applications. Two-step gelation The first binary system is composed of species α and β. The pathway to kinetic arrest is summarized in Fig. 1a as obtained with MD simulations. Initially the two-component mixture is equilibrated at high temperature, where it behaves as a one-component gas of hard spheres. A quench is then performed by suddenly lowering the temperature. At this stage, a short-range square-well (SW) attraction dominates between α-colloids, which form a gel coexisting with the β-gas. Finally, an identical SW attraction is activated between β-colloids, whose aggregates form in the confined environment imposed by the preexisting α-network. 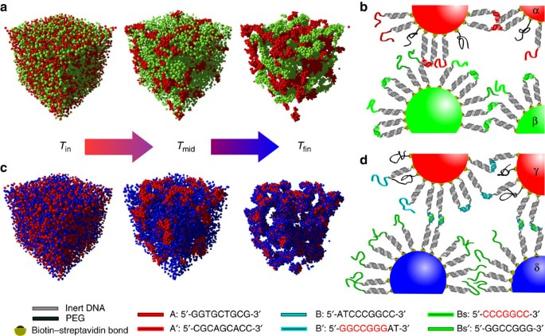Figure 1: Self-assembly pathway and experimental implementation of the two binary mixtures. (a) From left to right, snapshots for an MD simulation of the two-step gelation process of an α–β mixture. α- and β-particles are coloured in red and green, respectively. Initially, colloidal interactions are repulsive and the system equilibrates into a uniform gas phase. The α–α attraction is switched on, and gelation occurs. Finally, the β–β attraction is activated and the β-phase aggregates in the confined environment imposed by the α-template-gel. (b) Experimental implementation of the α- and β-particles with DNACCs. α–α and β–β hybridization interactions are activated at temperaturesTα>Tβsuch that the two-step aggregation pathway can be induced upon quenching fromTin>TαtoTα>Tmid>Tβand finally toTfin<Tβ. (c) From left to right, snapshots of an MD simulation of a core-shell gelation of a γ–δ mixture. γ-and δ-particles are coloured in red and blue, respectively. Initially, the γ–γ attraction is switched on, and forms a gel from the initially uniform gas phase. Upon activation of the γ–δ attraction, δ-particles coat the γ-gel as a single layer. δ–δ interactions are repulsive at every stage. (d) Experimental implementation of the γ–δ mixture with DNACCs. γ-colloids are functionalized withBandB′ sticky ends, giving rise to an intraspecies attraction forT<Tγ. δ-particles are coated only withBSsticky ends, complementary to part ofB′ (marked in red), such that a γ–δ attraction arises forT<Tδ<Tγ. The DNA constructs are grafted to the surface of the colloids via biotin–streptavidin bonds. To reduce the aggregation temperature of species α and γ, a fraction of the grafting sites is occupied by inert PEG polymers. Figure 1: Self-assembly pathway and experimental implementation of the two binary mixtures. ( a ) From left to right, snapshots for an MD simulation of the two-step gelation process of an α–β mixture. α- and β-particles are coloured in red and green, respectively. Initially, colloidal interactions are repulsive and the system equilibrates into a uniform gas phase. The α–α attraction is switched on, and gelation occurs. Finally, the β–β attraction is activated and the β-phase aggregates in the confined environment imposed by the α-template-gel. ( b ) Experimental implementation of the α- and β-particles with DNACCs. α–α and β–β hybridization interactions are activated at temperatures T α > T β such that the two-step aggregation pathway can be induced upon quenching from T in > T α to T α > T mid > T β and finally to T fin < T β . ( c ) From left to right, snapshots of an MD simulation of a core-shell gelation of a γ–δ mixture. γ-and δ-particles are coloured in red and blue, respectively. Initially, the γ–γ attraction is switched on, and forms a gel from the initially uniform gas phase. Upon activation of the γ–δ attraction, δ-particles coat the γ-gel as a single layer. δ–δ interactions are repulsive at every stage. ( d ) Experimental implementation of the γ–δ mixture with DNACCs. γ-colloids are functionalized with B and B ′ sticky ends, giving rise to an intraspecies attraction for T < T γ . δ-particles are coated only with B S sticky ends, complementary to part of B ′ (marked in red), such that a γ–δ attraction arises for T < T δ < T γ . The DNA constructs are grafted to the surface of the colloids via biotin–streptavidin bonds. To reduce the aggregation temperature of species α and γ, a fraction of the grafting sites is occupied by inert PEG polymers. Full size image The simulated two-step gelation is tested experimentally using a two-component mixture of fluorescently labelled DNA-coated polystyrene spheres with a diameter of 500 nm. These particles are used for all the experiments presented in this article. As shown in Fig. 1b , α-colloids are functionalized with a symmetric mixture (ratio 1:1) of double-stranded DNA (dsDNA) sequences terminated with single-stranded DNA (ssDNA) sticky ends A and A ′, complementary to each other. The use of dsDNA rigid spacers allows the sticky ends to explore a large volume around the grafting site and limits the entropic cost for hybridization [4] , [5] , [6] , [15] , [24] , [29] , [30] , [31] . Details of the DNA coatings are provided in the Methods section. Complementarity between ssDNA grafted on the same particle results in the formation of intra-colloidal loops and inter-colloidal bridges [15] , [29] , [30] , [31] . The latter are responsible for interspecies attraction between α-colloids, activated by quenching below the aggregation temperature T α ≈43 °C. Similarly to the α-species, β-colloids are coated with a symmetric mixture of complementary B S and B ′ S strands. The aggregation temperature between β-particles is T β ≈33 °C< T α . The two-step gelation is replicated by quenching the α–β mixture from the initial gas equilibrated at T in =55 °C, to an intermediate temperature T mid =40 °C, with T β < T mid < T α . At this stage, α-colloids undergo gelation, whereas β-colloids remain in the gas phase. After a percolating α-network is formed, we further decrease the temperature to T fin =25 °C< T β to induce gelation of the β-species. Epifluorescence microscopy snapshots of the three stages are shown separately for the two components in Fig. 2a . 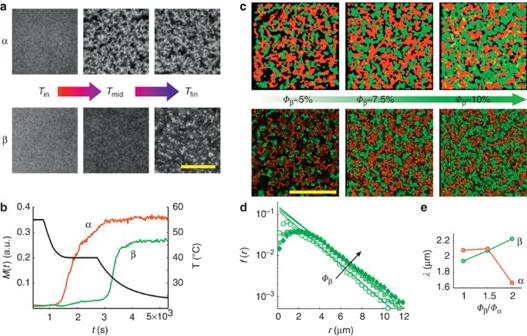Figure 2: Two-step gelation with DNACCs. (a) Epifluorescence snapshots of α- (top,) and β- (bottom) colloids at different stages of the quenching procedure for a sample withφα=φβ≈5%. Scale bar, 20 μm. (b) Evolution of temperature (black curve, right axis) andfor the two components (red curve for α, green curve for β, left axis) for a sample withφα≈5% andφβ≈10%. (c) Confocal fluorescence images of three arrested samples (bottom) and corresponding top view of 3D volume reconstructions (top) withφα≈5% and, from left to right,φβ≈5, 7.5 and 10% (α component in red, β component in green). Scale bar, 50 μm. (d) Chord-length distributions for the β-phase for samples shown inc. Circle symbols indicateφβ≈5%, square symbols indicateφβ≈7.5% and diamond symbols indicateφβ≈10%. Solid lines indicate exponential fits. (e) Persistence lengthλevaluated from chord-length distributions of α- and β-components for samples shown inc. Experiments with α–β mixtures were repeated five times, and for each sample, 30–50 confocal images of 91 × 91 μm2were taken at random positions within the samples. Figure 2: Two-step gelation with DNACCs. ( a ) Epifluorescence snapshots of α- (top,) and β- (bottom) colloids at different stages of the quenching procedure for a sample with φ α = φ β ≈5%. Scale bar, 20 μm. ( b ) Evolution of temperature (black curve, right axis) and for the two components (red curve for α, green curve for β, left axis) for a sample with φ α ≈5% and φ β ≈10%. ( c ) Confocal fluorescence images of three arrested samples (bottom) and corresponding top view of 3D volume reconstructions (top) with φ α ≈5% and, from left to right, φ β ≈5, 7.5 and 10% (α component in red, β component in green). Scale bar, 50 μm. ( d ) Chord-length distributions for the β-phase for samples shown in c . Circle symbols indicate φ β ≈5%, square symbols indicate φ β ≈7.5% and diamond symbols indicate φ β ≈10%. Solid lines indicate exponential fits. ( e ) Persistence length λ evaluated from chord-length distributions of α- and β-components for samples shown in c . Experiments with α–β mixtures were repeated five times, and for each sample, 30–50 confocal images of 91 × 91 μm 2 were taken at random positions within the samples. Full size image Our samples cannot be refractive-index matched because of the incompatibility of DNA with organic solvents. To allow high-quality optical imaging of opaque samples, we construct sample chambers in a slab geometry as sketched in Supplementary Fig. S1 [24] (ref.24). The activation of DNA-mediated attraction between micron-size colloids occurs within 1–2 °C across the aggregation temperature [4] , [7] , [32] . In our experiments, this temperature range is spanned in a few tens of seconds, much less than the time required for kinetic arrest, which is ~5 min. The activation of the attractive interactions can therefore be considered as instantaneous, consistent with our MD simulations protocol. DNA-mediated attraction is modelled in MD simulations with a SW potential, rather than a smoother profile. This is justified by the short range of the interactions, ~4% of the colloidal diameter, which makes the thermodynamic properties of the system independent of the details of the potential [33] , [34] . We monitor the evolution of both species via Fourier transform analysis of epifluorescence images taken separately for each component. We calculate the function I q ( t )=‹| J q ( t )| 2 ›/∫ J ( x , y )d x d y , where J q ( t ) is the two-dimensional Fourier transform of an epifluorescence image J ( x , y , t ), and ‹…› indicates a radial average. By assuming that intensity J ( x , y , t ) is proportional to the local density of one of the colloidal components, a two-dimensional structure factor can be obtained as S q ( t )= I q ( t )/| f q | 2 . The quantity | f q | 2 indicates a sort of ‘form factor’ that can be roughly estimated as , where is measured by averaging I q ( t ) over time while keeping the sample in the gas phase at T = T in . As demonstrated in Supplementary Fig. S2 , the function , develops a peak as soon as the aggregation is triggered [35] . The maximum amplitude grows monotonically in time until the kinetic arrest is reached. The maximum occurs at a wave vector q max that relates to the typical length scale of the aggregating structures as and shifts towards small wave vectors as the phase separation takes place [35] , [36] . The evolution of M ( t ) for the α–β mixture, shown in Fig. 2b , captures the formation sequence of the two-step gel. We obtain morphological information about the final arrested structures from confocal imaging. We produce three-dimensional (3D) reconstructions by processing confocal stacks with Gaussian filtering and thresholding algorithms. Further details on image processing are provided in the Methods section. Quantitative characterization is carried out by means of a chord-distribution analysis [36] , [37] , [38] . Chords are defined as the segments resulting from the intersection between straight lines and gel patterns on thresholded images (see Methods section, Supplementary Figs S3 and S4 ) [36] , [37] , [38] . Chord-length histograms f ( r ) show the exponential decay typical of patterns originating from arrested phase separation [36] . The decay length λ defines the persistence length of the structures [37] and provides a measure of the characteristic length scale of the arrested domains [36] . Colloidal structures formed by diffusion or reaction-limited aggregation, rather than by arrested phase separation, would exhibit a fractal morphology without a characteristic length scale. This would result in a power law rather than an exponential decay of f ( r ) [37] , [38] . The relative concentration of the two species has a tuning role for the morphology of the gels. In Fig. 2c , we show coexisting α–β gels with constant volume fraction for the α-phase φ α ≈5%, but increasing φ β ≈5, 7.5 and 10%. As expected, the morphology of the β-phase is influenced by the preexisting α-gel, which acts as a template for the β-aggregation. This influence is evident in the case of symmetric composition φ α = φ β , for which the β-species aggregates into disconnected clusters because of the confinement imposed by the α-gel. Such morphological asymmetry is confirmed by the chord-distribution length scales λ α > λ β , and is a direct consequence of the two-step kinetic arrest. In fact, binary mixtures in which the two components have an identical melting temperature form coexisting gels with identical morphology [24] (see Methods section and Supplementary Fig. S5 ). The domain size λ β grows upon increasing φ β to 7.5 and 10%, as shown in Fig. 2d . For the sample with φ β =2 φ α , we observe a significant drop in λ α , indicating that a high concentration of β-colloids in the initial gas phase inhibits the percolation of the α-component. Besides the confining effect of the α-gel, the morphology of the β-phase can be influenced by nonspecific α–β attraction that might result in the trapping of β-particles within the α-aggregates. Core-shell gelation By introducing controlled interspecies interactions mediated by DNA, we can further manipulate the structures and produce morphologies characterized by an even higher level of complexity. We exemplify this by presenting a second binary mixture composed of colloids γ and δ. The two-step arresting sequence is illustrated in Fig. 1c as obtained from MD simulations. After equilibrating the system at high temperature, we trigger the gelation of the γ-component by activating the γ–γ attraction, analogously to the two-step gelation. For the second step, we activate an interspecies γ–δ attraction while keeping the δ–δ interaction repulsive. This results in the formation of a single layer of δ-particles coating the percolating γ-gel, and producing a core-shell gel structure. Similarly to α-colloids, the γ DNACCs are functionalized with a symmetric mixture of complementary sticky ends B and B ′, which cause aggregation at temperature T < T γ ≈43 °C. Colloids δ are functionalized only with B S sticky ends, complementary to a sub-sequence of B ′ ( Fig. 1d ). Upon quenching to temperatures below T δ ≈33 °C, the specific γ–δ attraction is activated, triggering the formation of the shell. Because B S is not self-complementary, the δ–δ interaction remains repulsive. The two-step formation of core-shell gels is demonstrated by epifluorescence images in Fig. 3a and the evolution of the structure factor’s maximum, M ( t ), in Fig. 3b , for φ γ = φ δ ≈5%. We show a confocal image, and the corresponding 3D reconstruction from a similar sample in Fig. 3c , and a zoomed confocal stack in Supplementary Movie 1 . Also for the core-shell structures, the chord distribution provides quantitative morphological information as shown in Fig. 3d . We find a persistence length of the coating phase λ δ ≈570 nm, as expected, similar to the diameter of a single colloid. The persistence length of the total gels λ γ+δ is consistently larger than λ γ . 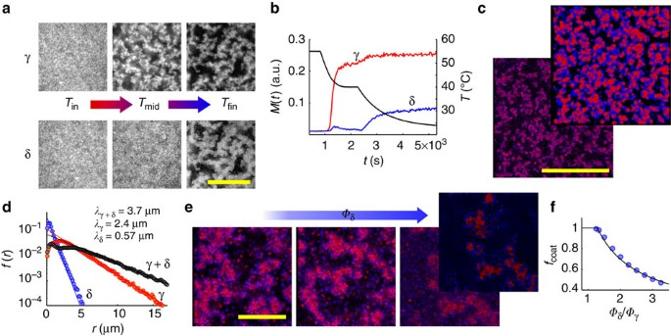Figure 3: Core-shell gels with DNACCs. (a) Epifluorescence snapshots of γ- (top) and δ- (bottom) colloids at different stages of the quenching procedure for a sample withφγ=φδ≈5%. Scale bar, 10 μm. (b) Evolution of temperature (black curve, right axis) andfor the two components (red curve for γ, blue curve for δ, left axis) for a sample withφγ=φδ≈5%. (c) Confocal image and corresponding 3D reconstruction for a sample withφγ=φδ≈5%. Scale bar, 50 μm. (d) Chord-length distribution calculated for the sample inc. Blue ? indicates the δ-phase, red ? indicates the γ-phase and grey ? indicates the total network obtained by adding up the δ- and γ-images. The lines are exponential fits. (e) Higher-magnification confocal images showing samples with constantφγ=5% and, from left to right,φδ=5, 7.5 and 10%. For the last sample, we show a time-averaged image to distinguish the δ-gas phase from the δ-shell surrounding the γ-core gel. Scale bar, 10 μm. (f) Fractionfcoatof δ-colloids adhering to the γ-gel as a function ofφδ/φγ. Symbols show simulation data, the black solid line is a fit with the modelfcoat(x)=(x−1+xc)−1+α, wherex=φδ/φγ,xc=1.29±0.03 andα=0.331±0.008. Experiments with γ–δ mixtures were repeated five times, and for each sample, 30–50 confocal images of 91 × 91 μm2were taken at random positions within the samples. Figure 3: Core-shell gels with DNACCs. ( a ) Epifluorescence snapshots of γ- (top) and δ- (bottom) colloids at different stages of the quenching procedure for a sample with φ γ = φ δ ≈5%. Scale bar, 10 μm. ( b ) Evolution of temperature (black curve, right axis) and for the two components (red curve for γ, blue curve for δ, left axis) for a sample with φ γ = φ δ ≈5%. ( c ) Confocal image and corresponding 3D reconstruction for a sample with φ γ = φ δ ≈5%. Scale bar, 50 μm. ( d ) Chord-length distribution calculated for the sample in c . Blue ? indicates the δ-phase, red ? indicates the γ-phase and grey ? indicates the total network obtained by adding up the δ- and γ-images. The lines are exponential fits. ( e ) Higher-magnification confocal images showing samples with constant φ γ =5% and, from left to right, φ δ =5, 7.5 and 10%. For the last sample, we show a time-averaged image to distinguish the δ-gas phase from the δ-shell surrounding the γ-core gel. Scale bar, 10 μm. ( f ) Fraction f coat of δ-colloids adhering to the γ-gel as a function of φ δ / φ γ . Symbols show simulation data, the black solid line is a fit with the model f coat ( x )=( x −1+ x c ) −1+ α , where x = φ δ / φ γ , x c =1.29±0.03 and α =0.331±0.008. Experiments with γ–δ mixtures were repeated five times, and for each sample, 30–50 confocal images of 91 × 91 μm 2 were taken at random positions within the samples. Full size image To further demonstrate that the δ–δ attraction is negligible and δ-colloids only form a single layer coating the surface of the γ-gel, we produce samples with increasing φ δ but constant φ γ ≈5%. High-magnification confocal images are shown in Fig. 3e , whose full size versions are shown in Supplementary Fig. S6 . For the case of φ δ =5%, the number of δ-colloids in the gas phase is similar to the number of γ-colloids. Both are compatible with a gas–gel coexistence. Increasing φ δ to ≈7.5%, we observe a clear growth of the number of free δ-colloids, indicating that the surface of the γ gel is saturated and further binding of the δ-particles is hindered. This saturation effect is more evident for samples with φ δ =10%, for which a time-averaged image is necessary to distinguish between the immobilized δ-particles making up the shell and the abundant δ-gas. We quantify the saturation effect with MD simulations by measuring the fraction f coat ( x ) of δ-colloids adhering to the γ-gel as a function of the relative composition x ≡ φ δ / φ γ , as shown in Fig. 3f . Experimental observation reveals that f coat ( x )<1 for x > x c , that is, non-adhering δ-colloids become observable beyond a threshold composition ratio slightly bigger than 1. By means of simulations, we obtain a more precise value x c =1.29±0.03, which is a fitted parameter of the simple power-law model f coat ( x )=( x −1+ x c ) −1+ α , with α =0.331±0.008. Multistep kinetic self-assembly enables further morphological manipulation by changing the timescale of the quench processes. We can process the same α–β or γ–δ mixtures with a very fast, one-step quench instead of the two-step quench. For the α–β mixture, this removes the morphological asymmetry, whereas the γ–δ mixture aggregates in a single binary gel. All the morphologies between this limiting situation and the ones obtained with two-step quenches are in principle accessible and will produce materials with different tunable properties. For example, a gas of core-shell clusters similar to that shown by Wu et al. [23] would emerge as a particular case in which, by shortening the waiting time between the two steps, the gelation of γ-colloids (first step) is blocked at the stage where the γ-clusters start to be covered by δ-colloids (second step). Colloidal structures assembled via DNA can be made permanent [30] , enabling a direct application of our strategy to the self-assembly of functional materials. For example, spongy phases generated in nature by arrested phase separation can produce structural colouring [18] , [19] , [20] , [21] . Similar materials may then be engineered based on our approach, with the additional possibility of tuning refractive-index contrast by having multiple components of different materials. In random lasers, amorphous assemblies of colloids are immersed in a medium that provides optical gain to ensure the multiple scattering required to reach the lasing threshold [39] . Resonant emission can be obtained by using randomly packed monodisperse spheres as scatterers [40] . Similarly, we suggest the use of colloidal gels with a controllable photonic response. Multiple components would also allow decoupling between the spatial distribution of the dyes providing gain, which can be incorporated in latex colloids [41] , and the scatterers. The manufacture of hybrid photovoltaics requires a controlled phase separation between conjugate polymers acting as light absorbers/donors and inorganic particles acting as acceptors [42] . Schemes analogous to our core-shell self-assembly could be adopted to build inorganic semiconductor scaffolds of different morphologies and coat them with organic particles. Furthermore, the thermal reversibility of the DNA interactions can be exploited to engineer responsive materials for sensing and drug release. As an example, consider the core-shell gels. The scaffold phase can be made of permanently bound inert colloids and covered with a shell of reversibly bound drug-filled nanoparticles [43] , [44] . Because of its porosity, the scaffold can be used to contain and deliver large and controllable quantities of drug-filled shell particles that can be released upon an external stimulus, such as a change in temperature or pH. We conclude by emphasizing that our strategy is not limited to the use of DNA. Supramolecular chemistry provides a wide range of tags with selective interactions [45] , [46] , the functionality of which is not limited to physiological environments as it is for DNA. Summarizing, we introduce an alternative means of controlling the self-assembly of colloidal particles into amorphous materials. Contrary to equilibrium self-assembly strategies, in which the target configuration is only determined by equilibrium interactions between the building blocks, our approach relies on both the selectivity of DNA interactions and their sequential activation to induce multistep kinetic arrest and tune the morphology of the final configuration. We describe two model systems to demonstrate the potential and flexibility of our scheme. The first is a two-component mixture undergoing a two-step gelation, with the second colloidal species forced to gel in the confined environment produced by the first aggregating species. The second system self-assembles in a core-shell colloidal gel, with the first-formed network acting as a scaffold and the second component forming a shell around it. Multistep kinetic self-assembly of mesoscopic building blocks mediated by selective interactions (as for DNA) holds great promise as a general approach for reliable self-assembly of mesoporous materials. Computer simulations Event-driven MD simulations are performed in cubic boxes with periodic boundary conditions. The colloids are modelled by means of a SW potential, with a hard-sphere core and a well whose depth is either set equal to ∈ ij =− ∈ 0 , when the i and j species are attractive, or to ∈ ij =0, when they are considered as repulsive. The simulations involve up to 2 × 10 4 particles. The colloids have equal diameter σ =1 and equal mass m =1. The potential is chosen to be short-ranged, that is, 3% of the diameter. We use reduced units, that is, k B =1 and ∈ 0 =1. The quenches are performed by lowering the temperature from T =100 to the final value T =0.05, well below the known critical temperature T c =0.3 for a single-component system [47] . As the system falls out of equilibrium, averages over 10 independent realizations of the initial conditions are considered instead of time averages. DNA coatings and sample preparation DNA (Integrated DNA Technology) is grafted to streptavidin-coated colloids via biotin–streptavidin linkage. The structure of the DNA constructs is: biotin–5′-TTTTT–dsDNA spacer–TTTTT–ssDNA sticky end-3′. The dsDNA spacer has a length of 60 bp. The 5-thymine sequences are added to confer more flexibility. The constructs are prepared before being grafted to the colloids by hybridizing two ssDNA strands: (i) biotin–5′-TTTTT– S –TTTTT–sticky end-3′ and (ii) S ′. The sequence of the ssDNA S is 5′-GAGGAGGAAAGAGAGAAAGAAGGAGAGGAGAAGGGAGAAAAGAGAGAGGGAAAGAGGGAA-3′. The sequence S ′ is complementary to S . Strands (i) and (ii) are mixed in 10 mM Tris-EDTE buffer (TE; Sigma Aldrich), heated up to 80 °C for 2 h and left to cool down overnight to allow hybridization of S and S ′ sequences. We use a (i)/(ii) concentration ratio equal to 1/2 to guarantee complete hybridization of the (i) constructs. The sequences of the sticky ends are as follows: A : 5′-GGTGCTGCG-3′; A ′: 5′-CGCAGCACC-3′; B : 5′-ATCCCGGCC-3′; B ′: 5′-GGCCGGGAT-3′; B S : 5′-CCCGGCC-3′; and B S ′: 5′-GGCCGGG-3′. The melting temperatures of the free sticky ends in solution are: B – B ′: 37.5 °C, A – A ′: 37.8 °C and B S – B S ′( B ′): 30.2 °C, calculated at 50 mM ionic strength and 0.25 μM oligonucleotide concentration. Streptavidin-coated polystyrene colloids with diameter of 500 nm and biotin-binding capacity of ~500 pmol mg −1 are purchased from Microparticles GmbH (Berlin). To distinguish different components, the particles are fluorescently labelled with dyes FluoGreen (492/519 nm) and FluoRed (530/607 nm). The coating is carried out by dispersing the colloids in a TE solution containing a mixture of DNA constructs and (eventually) biotin-labelled polyethylene glycol (5000MW PEG; Laysan Bio Inc., Arab, AL, USA). The inert polymer is used to reduce the DNA-coating density and tune the aggregation temperature. The compositions of the DNA mixtures used to coat the four colloidal species are: α: A (2.5 × )+ A ′ (2.5 × )+PEG (0.3 × ); β: B S (2.5 × )+ B S ′ (2.5 × ); γ: B (2.5 × )+ B ′ (2.5 × )+PEG (0.3 × ); and δ: B S (5 × ). In brackets, we report the amount of DNA and PEG expressed in units of the total binding capacity of the colloids, that is, 2.5 × indicates a 2.5 times excess compared with the total binding capacity of the colloids. To allow the binding, the mixtures of DNA and colloids contained in a plastic vial are left for 2 h at room temperature. We carry out a washing protocol to remove unbound molecules. We dilute the solutions up to a volume of 600 μl and heat up to 45 °C for 5 min to melt colloidal aggregates forming in α-, β- and γ-samples (at the low ionic strength of TE buffer, the aggregation temperature of all species is <45 °C). To maintain the same experimental conditions, the heating step is performed also for δ-samples, even though δ–δ interactions are repulsive. Afterwards, we centrifuge the vials and replace 400 μl of solution with the same amount of clean TE buffer kept at 45 °C. This washing cycle is repeated 10 times. Finally, we pellet the samples once more, remove all the buffer and re-suspend the colloids into an appropriate quantity of density-matched TE buffer. The density-matched TE buffer is prepared by adding 50 mM NaCl and dissolving sucrose to match the density of polystyrene (1.05 g cm −3 ). To allow high-quality imaging of opaque samples, we construct sample chambers with a slab geometry. See Supplementary Fig. S1 for a schematic of the chamber. α–β and γ–δ mixtures are prepared before injecting them into the chambers by mixing appropriate quantities of the single components, depending on the required concentration ratio. The total volume of the mixture at this stage is 8 μl. We add 1 μl of 0.2 mM biotin solution. The biotin saturates all the free binding sites that could be potentially occupied by freely diffusing DNA strands, which would give rise to undesired interactions. The samples are heated up for 2–3 min at 60 °C, then mixed to obtain a uniform composition, and then 6 μl are injected into a pre-heated chamber, which is immediately sealed to avoid any evaporation. Thermal processing Thermal processing is performed on a Nikon Eclipse Ti-E inverted microscope while imaging using a Plan Apo VC × 20/0.75 or Plan Fluor × 40/0.75 dry objectives. The samples are heated up using a copper heating block, and the temperature is monitored with a thermocouple in contact with the chamber. We leave all the mixtures at T in =55 °C for ~30 min to allow equilibration of the gas phase, and then we let the system cool down to T mid =40 °C, wait for the α- or γ-gels to form and further cool down to T fin ~25 °C. We monitor the two-step quenching by taking epifluorescence snapshots at intervals of 30 s. Once T fin is reached, the samples are moved to a Leica TCS SP5 microscope equipped with an HCX PL APO CS × 100/1.4 oil immersion objective for confocal imaging. Image analysis For each sample, the chord distribution is measured from 40–50 confocal stacks taken at random locations. From each stack, we select the single confocal image corresponding to the middle of the sample (see Supplementary Movie 2 for a full stack). This is done by selecting the image for which the integrated intensity H ( z )=∫ I ( x , y , z )d x d y is maximum. The selected confocal slice ( Supplementary Fig. S3a ) is processed with a Gaussian filter ( Supplementary Fig. S3b ), then thresholded to obtain a binary image ( Supplementary Fig. S3c ). To allow for a meaningful comparison, the threshold is determined with the same criterion for all α–β mixtures. We consider separately the two fluorescent channels for each image and threshold them with an underestimated threshold value, then we measure the fraction of pixels in which the α- and β-binary images overlap. We iterate this process increasing the threshold value until the fraction of pixels in which α- and β-binary images overlap becomes <3%. For γ–δ mixtures, this criterion overestimates the threshold value, which is instead calculated using Otsu’s method [48] (matlab built-in function). Chord distributions are calculated by drawing a set of straight lines on the binary images. The intersections between the lines and of the two components are then measured and sampled to obtain histograms f ( r ) of the chord-length distributions ( Supplementary Fig. S4a ). For each image, we use a regularly spaced grid of straight lines directed along the x and y directions. Given that our samples are amorphous and have no preferential orientation, this choice does not bias the results. The distributions f ( r ) show an exponential tail that identifies the lengthscale λ , a measure of the persistence length of the branched structures [37] , [38] . λ has been recently identified as a good parameter to characterize the morphology of arrested colloidal phases [36] . As shown in Supplementary Fig. S4b , it is also possible to calculate f ( r ) for the overall gel structure and the network of pores surrounding the gels. Two-step versus one-step gelation To demonstrate how the pre-formed α-network affects the morphology of the β-gel in a two-step gelation experiment, we compare an α–β sample ( φ α = φ β ≈5%) with an α–γ sample ( φ α = φ γ ≈5%). Because T α ≈ T γ ≈43 °C, upon quenching, α- and γ-components undergo gelation at the same time [24] . As demonstrated with 3D reconstructions in Supplementary Fig. S5 , the morphology of the α–β and α–γ gels is visibly different. In particular in the two-step sample, the β-component forms a cluster phase embedded within the α-network, whereas in the case of one-step gelation, both α- and γ-components form interpenetrating networks. This is quantified by a chord-distribution analysis. In fact, for the α–β sample, we find λ α =2.1 μm > λ β =1.9 μm, whereas for the α–γ sample, we find λ α = λ γ =2.1 μm. How to cite this article: Di Michele, L. et al. Multistep kinetic self-assembly of DNA-coated colloids. Nat. Commun. 4:2007 doi: 10.1038/ncomms3007 (2013).